Neural progenitor cells orchestrate microglia migration and positioning into the developing cortex Microglia are observed in the early developing forebrain and contribute to the regulation of neurogenesis through still unravelled mechanisms. In the developing cerebral cortex, microglia cluster in the ventricular/subventricular zone (VZ/SVZ), a region containing Cxcl12-expressing basal progenitors (BPs). Here we show that the ablation of BP as well as genetic loss of Cxcl12 affect microglia recruitment into the SVZ. Ectopic Cxcl12 expression or pharmacological blockage of CxcR4 further supports that Cxcl12/CxcR4 signalling is involved in microglial recruitment during cortical development. Furthermore, we found that cell death in the developing forebrain triggers microglial proliferation and that this is mediated by the release of macrophage migration inhibitory factor (MIF). Finally, we show that the depletion of microglia in mice lacking receptor for colony-stimulating factor–1 (Csf-1R) reduces BPs into the cerebral cortex. The germinal niche of the developing cerebral cortex consists of two distinct mitotically active populations of cells: radial glial cells (RGs) of the ventricular zone (VZ) and basal progenitors (BP) of the Subventricular zone (SVZ) [1] . BPs originate from asymmetric cell divisions of RG and are fated to differentiate into cortical plate excitatory neurons [2] , [3] and to regulate inhibitory neurons’ migration through the release of the chemokine Cxcl12. The downregulation of the transcription factor Tbr2 impairs BP generation and induces a significant reduction of Cxcl12 into the SVZ [4] that, in turn, affects inhibitory neurons migration [5] , [6] . Accordingly, inhibitory neurons lacking CxcR4 —that is one of the two Cxcl12 receptors [7] , [8] —are impaired in their homing into the cerebral cortex [9] , while CxcR7 is involved in the regulation of CxcR4 protein levels [10] . Microglia are immune-relevant cells of the central nervous system that are generated within the yolk sac at embryonic day (E) 8 and colonize the forebrain just before the onset of neurogenesis [11] , [12] . Once seeded into the cerebral cortex, microglia first accumulate at the pail surface and into the choroid plexus and then penetrate the cortical wall, clustering into a restricted laminar band that overlaps the cortical VZ/SVZ [13] , [14] , [15] . To date, little is known about mechanisms regulating microglia migration, recruitment and positioning into the developing cortex. However, since the ability of microglia to colonize cortical VZ/SVZ is conserved among species (that is, rodents, monkeys and humans) [14] , it is reasonable to hypothesize that also the molecular mechanism/s controlling their recruitment and function are well conserved along evolution. Using conditional and no conditional transgenic mice and in uteri electro oration techniques, here we show that BP, through the secretion of Cxcl12, drive CxcR4 - and CxcR7 -expressing microglia to cluster into the VZ/SVZ of the developing cerebral cortex. A finding supported by the fact that we found a profound alteration of microglia cell number and positioning within the developing cortex in transgenic mice in which neurogenesis was defective and the number of BP was consistently reduced. A further confirmation of this bidirectional axis is that the lack of the receptor for colony-stimulating factor-1 (Csf-1R), impairing microglia development, causes a significant depletion of BP into the cerebral cortex. We also found that microglia heavily proliferate in the presence of massive neural progenitor cell death—as that occurring in mice electro orated with the suicide gene thymidine kinase—in order to efficiently phagocytose dead cells. This process is molecularly orchestrated by macrophage migration inhibitory factor (MIF) released into the VZ/SVZ by RG cells. Altogether, our data indicate the presence of a bidirectional cross-talk between neural precursors (both BP and RG) and microglia in the developing cortex. This cross talk—sustained by a chemokine–chemokine receptor axis—is necessary to regulate neurogenesis in order to protect the developing cortex from unexpected and unfavourable damage. Cxcl12 mediates microglia recruitment into the VZ/SVZ We analysed cortical microglia at different time points during embryonic development (E10.5, E14.5, E16.5 and E18.5) in wild-type (WT) C57Bl/6 and in Cx3cR1-GFP (green fluorescent protein) transgenic mice [16] , in which microglia are fluorescent. We found that virtually all Cx3cR1-GFP + or F4/80 + cells scored at E15.5 and E18.5 co-expressed Iba1 ( Supplementary Fig. 1a,b ), suggesting that these markers can be used interchangeably to label microglia. While at E10.5 the vast majority of Iba1 + cells were located within the meninges ( Fig. 1a,b ), at E14.5, E16.5 and E18.5 such cells were preferentially clustered into the VZ/SVZ of the cerebral cortex ( Supplementary Fig. 1a–c ) [15] . Because microglia cell number significantly increased along neurogenesis in cortical and subcortical areas ( Fig. 1c,d ), we hypothesized the existence of a functional relationship between neurogenesis and microglia accumulation into the developing cerebral cortex. We focused on Tbr2 + BP cells, a population of intermediate neuronal progenitor cells preferentially positioned in the SVZ—the area where microglia accumulates during brain development—and known to express the chemoattractant molecule Cxcl12 ( Fig. 1e–g ) [17] , [18] . We found that microglia were greatly enriched in regions, such as the cortical–striatal notch and the dentate gyrus of the forebrain, where we concomitantly found that Cxcl12 was highly expressed ( Fig. 1h ). Similar results were obtained in the human developing forebrain, as we observed IBA1 + microglia preferentially confined in regions where both CXCL12 and TBR2 were expressed in 7- and 20-week-old human fetal brains ( Supplementary Fig. 2a–f ). 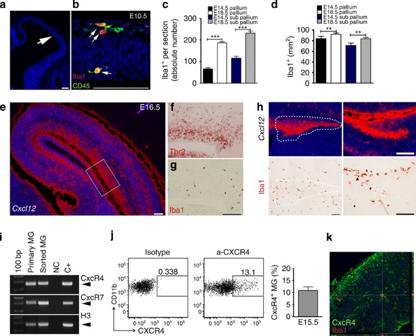Figure 1: Microglia distribution into the cerebral cortex overlaps Cxcl12+cortical domains. (a) Low magnification of the cerebral cortex at E10.5. High magnification (arrow) is shown inb(n=3). Labelling for Iba1 and CD45 in the cortical wall shows double-positive cells in the cortex and in the meninges (arrows indicate Iba1/CD45+cells). (c,d) Absolute numbers and cell densities of Iba1+cells were calculated by stereology at E14.5 and E18.5, and means±s.e.m. (pallium indicates the cerebral cortex and the hippocampus, while the sub pallium indicates basal ganglionic eminences and the septum,n=6 for each group). (e) Representative E16.5 cortical section probed forCxcl12, boxed area indicates the VZ/SVZ of the lateral cerebral cortex. (f,g) High magnification sections labelled for Tbr2 and Iba1 (n=5). (h) Cxcl12+and Iba1+cell distribution at the corticostriatal boundary and into the Dentate Gyrus at E16.5 (n=5). (i) Representative RT–PCR forCxcR7,CxcR4and the housekeeping geneH3performed on P2 brain-derived primary microglia cell culture (primary MG) and on E15.5-sorted CD45low/CD11b+cells (sorted MG;n=3 independent experiments). (j) Representative plot of CxcR4+cells, gated on CD45+CD11b+Ly6c−cells from E15.5 brains (n=3 independent experiments). (k) Double labelling for Iba1 and CxcR4 in the cortical wall of E15.5 brain. Scale bar represents 100 μm. A two-tailedt-test was used to assess statistical significance: **P<0.01, ***P<0.001. Figure 1: Microglia distribution into the cerebral cortex overlaps Cxcl12 + cortical domains. ( a ) Low magnification of the cerebral cortex at E10.5. High magnification (arrow) is shown in b ( n =3). Labelling for Iba1 and CD45 in the cortical wall shows double-positive cells in the cortex and in the meninges (arrows indicate Iba1/CD45 + cells). ( c , d ) Absolute numbers and cell densities of Iba1 + cells were calculated by stereology at E14.5 and E18.5, and means±s.e.m. (pallium indicates the cerebral cortex and the hippocampus, while the sub pallium indicates basal ganglionic eminences and the septum, n =6 for each group). ( e ) Representative E16.5 cortical section probed for Cxcl12 , boxed area indicates the VZ/SVZ of the lateral cerebral cortex. ( f , g ) High magnification sections labelled for Tbr2 and Iba1 ( n =5). ( h ) Cxcl12 + and Iba1 + cell distribution at the corticostriatal boundary and into the Dentate Gyrus at E16.5 ( n =5). ( i ) Representative RT–PCR for CxcR7 , CxcR4 and the housekeeping gene H3 performed on P2 brain-derived primary microglia cell culture (primary MG) and on E15.5-sorted CD45 low /CD11b + cells (sorted MG; n =3 independent experiments). ( j ) Representative plot of CxcR4 + cells, gated on CD45 + CD11b + Ly6c − cells from E15.5 brains ( n =3 independent experiments). ( k ) Double labelling for Iba1 and CxcR4 in the cortical wall of E15.5 brain. Scale bar represents 100 μm. A two-tailed t -test was used to assess statistical significance: ** P <0.01, *** P <0.001. Full size image To determine whether Cxcl12 might contribute to Iba1 + cell recruitment into the VZ/SVZ, we examined the expression of the Cxcl12 receptors CxcR4 and CxcR7 on microglia [19] , [20] . Ex vivo CD45 low /Cd11b + -sorted cells from E15.5 brains, as well as primary microglia cell cultures generated from P2 brains, expressed both receptors at robust levels ( Fig. 1i ). Flow cytometry-mediated analysis of CD45 + /Cd11b + /Ly6C − cells from E15.5 cortices showed that ~13% of them were also positive for CxcR4 ( Fig. 1j ). Accordingly, Iba1 + /CxcR4 + double-positive cells were found in the SVZ at E14.5 ( Fig. 1k ). To verify whether Cxcl12 + BPs influence microglia number and positioning into the VZ/SVZ, we unilaterally electroporated in utero plasmids coding for Cxcl12 and GFP at E14.5 ( Fig. 2a–c ). 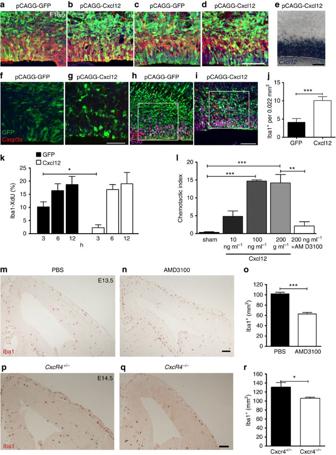Figure 2: The overexpression of Cxcl12 recruits microglia into the VZ/SVZ. Confocal images of E16.5 cortices receiving GFP plasmids (a,c,f,h) or GFP/Cxcl12 plasmids (b,d,e,g,i). (a,b) Double labelling for Blbp, GFP. (c,d) Double labelling for Tbr2 and GFP. (e) EctopicCxcl12expression in the VZ/SVZ of Cxcl12-electroporated brains (n=5 for each group). (f,g) Distribution of Casp3a in GFP and GFP/Cxcl12-electroporated brains. (h,i) Confocal images of GFP (green), EdU (violet) and Iba1(red) in electroporated embryos pulsed with EdU for 3 h before killing. (j) Iba1+cells (means±s.e.m.) and Iba1/XdU+cells (percentages±s.e.m.) in boxed areas (k;n=5 brains for each group). (l) Chemotactic responses of primary microglia to increasing amount of Cxcl12 and its reversion by AMD3100 (n=3). (m,n) Iba1 detection in E13.5 coronal sections from brains injected either with PBS (m) or AMD3100 (n). Cell counts (mean±s.e.m) are provided ino, (n=3 brains for each group). (p,q) Iba1+cells in E14.5 coronal sections from CxcR4+/−and from CxcR4−/−brains and their means±s.e.m. inr(n=3 brains for each group). Scale bar represents 100 μm. A two-tailedt-test was used to assess statistical significance: *P<0.05, **P<0.01, ***P<0.001. The overexpression of GFP and Cxcl12 in RG (Blbp + cells) and BP (Tbr2 + cells) of the VZ and SVZ did not affect cell morphology, while efficiently increased Cxcl12 levels ( Fig 2a–e ). Further, increased levels of Cxcl12 in the VZ/SVZ did not affect cell survival of RG and BP ( Fig 2f,g ) but increased the number of Calbindin + (CaB) interneurons in the SVZ ( Supplementary Fig. 3a,b ) [5] , and, above all, the number ( Fig 2h–j )—but not the proliferation ( Fig. 2k )—of microglia in the VZ/SVZ. Accordingly, we showed that in vitro primary microglia were capable of responding to Cxcl12-mediated chemotactic signal. This response was completely abolished by administering the antagonist of CxcR4, AMD3100 (ref. 21 ; Fig. 2l ). We did exclude that our results could be biased by any procedure related to nonspecific inflammatory reaction by assessing the absence of pro-inflammatory cytokine transcripts ( IL-1β (interleukin-1β) , TNF-α (tumour-necrosis factor-α) and IFN-γ (interferon-γ) ) in the brain of embryos receiving GFP and Cxcl12 plasmids ( Supplementary Fig. 4 ). To further confirm the chemoattractant properties of Cxcl12, we injected AMD3100 (1 μl, 12.6 mM) into the lateral ventricle of E12.5 embryos. Twenty hours after the injection, treated embryos showed a significant reduction in Iba1 + cells in both cerebral cortex and basal ganglionic eminences ( Fig. 2m–o ). A similar depletion of microglia number was also observed in E14.5 CxcR4 −/− cortices ( Fig. 2p–r ). Likewise, E16.5 Gfap Cre Cxcl12 flox/flox mice, while showing substantial downregulation of Cxcl12 in the SVZ ( Supplementary Fig. 2c,d ) also displayed a significant reduction of microglia ( Supplementary Fig. 2e–g ) and SVZ-confined CaB + interneurons in the developing cerebral cortex ( Supplementary Fig. h,i ). These results indicate that the blockage of Cxcl12/CxcR4 interaction is per se sufficient to inhibit microglia cell homing into the SVZ. Figure 2: The overexpression of Cxcl12 recruits microglia into the VZ/SVZ. Confocal images of E16.5 cortices receiving GFP plasmids ( a , c , f , h ) or GFP/Cxcl12 plasmids ( b , d , e , g , i ). ( a , b ) Double labelling for Blbp, GFP. ( c , d ) Double labelling for Tbr2 and GFP. ( e ) Ectopic Cxcl12 expression in the VZ/SVZ of Cxcl12-electroporated brains ( n =5 for each group). ( f , g ) Distribution of Casp3a in GFP and GFP/Cxcl12-electroporated brains. ( h , i ) Confocal images of GFP (green), EdU (violet) and Iba1(red) in electroporated embryos pulsed with EdU for 3 h before killing. ( j ) Iba1 + cells (means±s.e.m.) and Iba1/XdU + cells (percentages±s.e.m.) in boxed areas ( k ; n =5 brains for each group). ( l ) Chemotactic responses of primary microglia to increasing amount of Cxcl12 and its reversion by AMD3100 ( n =3). ( m , n ) Iba1 detection in E13.5 coronal sections from brains injected either with PBS ( m ) or AMD3100 ( n ). Cell counts (mean±s.e.m) are provided in o , ( n =3 brains for each group). ( p , q ) Iba1 + cells in E14.5 coronal sections from CxcR4 +/− and from CxcR4 −/− brains and their means±s.e.m. in r ( n =3 brains for each group). Scale bar represents 100 μm. A two-tailed t -test was used to assess statistical significance: * P <0.05, ** P <0.01, *** P <0.001. Full size image BPs expressing Cxcl12 drive the positioning of microglia within the developing brain Since the genetic ablation of Tbr2 greatly reduces Cxcl12 levels into the VZ/SVZ [5] , we generated Gfap Cre /Tbr2 flox/flox mice in order to eliminate Tbr2 expression in the cerebral cortex and to assess microglia cell positioning and number ( Fig. 3a,b ). In agreement with previous data [5] , Cxcl12 was greatly reduced in E16.5 Gfap Cre /Tbr2 flox/flox mice ( Fig. 3c,d ). This reduction was associated with a significant decrease in cortical microglia ( Fig. 3e–g ). Since the overexpression of Tbr2 in RG increases BP number and Cxcl12 expression [4] , we next assessed whether the overexpression of Tbr2 might trigger microglia accumulation into the VZ/SVZ. We electroporated plasmids encoding Tbr2 and GFP at E14.5, and brains were probed for Cxcl12 2 days later, at E16.5. While the overexpression of Tbr2 significantly augmented Cxcl12 levels in the VZ/SVZ, the overexpression of the GFP control plasmid did not alter these levels ( Fig. 3h ). In Tbr2 overexpressing mice we found an overall increase of microglia in the VZ/SVZ ( Fig. 3i–k ); however, we did not find any difference in the number of the Iba1/EdU + proliferating cells ( Fig. 3l ). 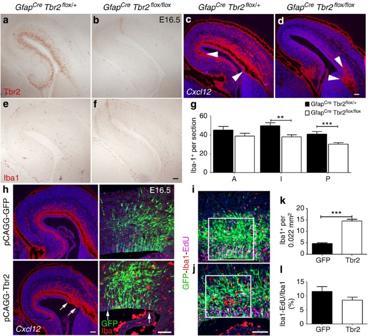Figure 3: Tbr2 regulates microglia influx into the cortical VZ/SVZ. E16.5GfapCreTbr2flox/+(a,c,e) andGfapCreTbr2flox/flox(b,d,f) coronal sections; (a,b)Tbr2labelling, (c,d)Cxcl12expression byin situhybridization, (e,f) distribution of Iba1+cells. (g) Iba1+cell quantifications (means±s.d.) at three different cortical levels along the anterior–posterior axis (A: anterior, I: intermediate and P: posterior;n=3 for each group). (h) E16.5 cerebral cortices electroporated either with GFP or GFP/Tbr2 plasmids probed forCxcl12to identify the ectopic expression ofCxcl12in the VZ/SVZ (arrow in left panel indicates the electroporated region). (h) Parallel sections probed for GFP and Iba1. (i,j) Electroporated embryos pulsed with EdU for 3 h before being killed and labelled for GFP, Iba1 and EdU. (k) Iba1+cell quantifications (means±s.e.m.) in boxed areas (n=5 for each group). (l) Iba1/EdU+cells (percentages±s.e.m.) in boxed areas (n=4 for each group). Scale bar represents 100 μm. A two-tailedt-test was used to assess statistical significance: **P<0.01, ***P<0.001. Figure 3: Tbr2 regulates microglia influx into the cortical VZ/SVZ. E16.5 Gfap Cre Tbr2 flox/+ ( a , c , e ) and Gfap Cre Tbr2 flox/flox ( b , d , f ) coronal sections; ( a , b ) Tbr2 labelling, ( c , d ) Cxcl12 expression by in situ hybridization, ( e , f ) distribution of Iba1 + cells. ( g ) Iba1 + cell quantifications (means±s.d.) at three different cortical levels along the anterior–posterior axis (A: anterior, I: intermediate and P: posterior; n =3 for each group). ( h ) E16.5 cerebral cortices electroporated either with GFP or GFP/Tbr2 plasmids probed for Cxcl12 to identify the ectopic expression of Cxcl12 in the VZ/SVZ (arrow in left panel indicates the electroporated region). ( h ) Parallel sections probed for GFP and Iba1. ( i , j ) Electroporated embryos pulsed with EdU for 3 h before being killed and labelled for GFP, Iba1 and EdU. ( k ) Iba1 + cell quantifications (means±s.e.m.) in boxed areas ( n =5 for each group). ( l ) Iba1/EdU + cells (percentages±s.e.m.) in boxed areas ( n =4 for each group). Scale bar represents 100 μm. A two-tailed t -test was used to assess statistical significance: ** P <0.01, *** P <0.001. Full size image On the whole, our results indicate that Cxcl12 -expressing BPs play a relevant role in directing microglia into the SVZ. Since it has been previously shown that the inhibition of the canonical Notch signalling in the developing forebrain might cause the premature differentiation of RG into neurons [22] , [23] , [24] , [25] , we then asked whether the blockage of Delta/Notch signalling into the developing cortex could lead to an overproduction of BP that, in turn, might alter microglia number and/or positioning within the cerebral cortex. Thus, to induce blockage of Notch signalling in cortical RG, we electroporated E14.5 forebrains with a plasmid carrying the dominant-negative form of Mastermind-like 1 gene ( dnMAMl ) [26] . The overexpression of dnMAMl plasmids induced an increase in the number of GFP + cells into the SVZ, the region in which BPs are normally residing, and a decrease in GFP + cells into the VZ, where RGs are normally located ( Fig. 4a,b,g,h ). Accordingly, dnMAMl electroporation increased the relative number of GFP + Tbr2 + BP in the cortex, as shown in constructed laminar bins encompassing germinal niches ( Fig. 4a–d ). Coherently, the number of phospho-histone H3 + (pH3) mitoses into the SVZ was significantly increased in mice receiving the dnMAMl plasmid ( Fig. 4e ). The overexpression of dnMAMl dramatically increased Cxcl12 levels into the SVZ ( Fig. 4f ) and the number ( Fig. 4g–i )—but not the proliferation ( Fig. 4j )—of microglia in the same areas. Of note, dnMAML plasmids injected into E14.5 Gfap Cre Cxcl12 flox/flox brains did not increase the number of Iba1 + cells, further confirming that Cxcl12 is necessary to drive microglia accumulation in the SVZ ( Fig. 4k,l ). Interestingly, the overexpression of dnMAMl also increased the number of Iba1 + cells floating into the ventricular cavity of the forebrain ( Supplementary Fig. 5a,b ); these latter cell population exhibited round cell morphology and were often organized in clusters around the Transthyretin ( Ttr ) + choroid plexus cells ( Supplementary Fig. 5d,e ) [27] . Accumulation of Iba1 + cells into the ventricular cavity was also seen in embryos receiving the overexpression of Cxcl12 , but not in embryos receiving GFP plasmids ( Supplementary Fig. 5a,b ). We also confirmed that cortices electroporated with dnMAMl did not express pro-inflammatory cytokines ( Supplementary Fig. 4 ) or CD206—a receptor mediating the phagocytosis of intracellular pathogens [28] ( Supplementary Fig. 6 )—thus ruling out possible adverse effects related to embryo manipulation and injection procedures. 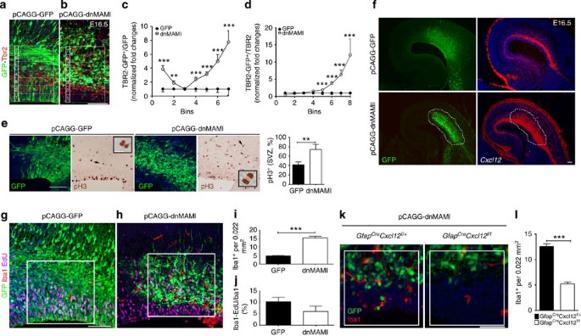Figure 4: Delta/Notch blockage increases microglia in the cerebral cortex. (a,b) E16.5 cortical sections electroporated either with GFP (a) or with GFP/dnMAMl (b) labelled for GFP and Tbr2. Tbr2+cells were counted in sectors 200 μm wide, subdivided into bins of 30 μm in height that were numbered from 1–7. (c) Quantification of Tbr2/GFP+cells over the total number of GFP+cells (normalized fold changes±s.e.m.). (d) Quantification of Tbr2/GFP+cells over the total number of Tbr2+cells (normalized fold changes± s.e.m.;n=6 brains for each group). (e) GFP and pH3 labelling in embryos receiving GFP or GFP/dnMAMl plasmids. Insets are showing high magnifications of SVZ-confined pH3+mitoses, histogram on the left shows quantifications of pH3+cells (percentages±s.d.;n=6 brains for each group). (f) Adjacent sections from embryos receiving GFP or GFP/dnMAMl labelled for GFP andCxcl12. Low magnification indicates localizations of GFP+patches. Dotted areas infindicate GFP patches in GFP/dnMAMl-electroporated brains displaying high levels ofCxcl12mRNA (n=6 for each group). (g,h) GFP, EdU and Iba1 labelling in electroporated embryos injected with EdU (3 h). Boxed areas indicate the region of interest in electroporated patches from GFP (g) and GFP/dnMAMl (h) embryos. (i) Quantifications of Iba1+cells (mean±s.e.m.,n=7 brains for each group), while percentages±s.e.m. of Iba1/EdU+cells are provided inj(n=5 for each group). (k) Total number of Iba1+cells in GFP/dnMAMl-electroporated patch performed onGfapCreCxcl12f/+andGfapCreCxcl12f/fmice, while quantifications are shown inl(means±s.e.m.,n=3 for each group). Scale bar represents 100 and 10 μm for insets ine. A two-tailedt-test was used to assess statistical significance: **P<0.01, ***P<0.001. Figure 4: Delta/Notch blockage increases microglia in the cerebral cortex. ( a , b ) E16.5 cortical sections electroporated either with GFP ( a ) or with GFP/dnMAMl ( b ) labelled for GFP and Tbr2. Tbr2 + cells were counted in sectors 200 μm wide, subdivided into bins of 30 μm in height that were numbered from 1–7. ( c ) Quantification of Tbr2/GFP + cells over the total number of GFP + cells (normalized fold changes±s.e.m.). ( d ) Quantification of Tbr2/GFP + cells over the total number of Tbr2 + cells (normalized fold changes± s.e.m. ; n =6 brains for each group). ( e ) GFP and pH3 labelling in embryos receiving GFP or GFP/dnMAMl plasmids. Insets are showing high magnifications of SVZ-confined pH3 + mitoses, histogram on the left shows quantifications of pH3 + cells (percentages±s.d. ; n =6 brains for each group). ( f ) Adjacent sections from embryos receiving GFP or GFP/dnMAMl labelled for GFP and Cxcl12 . Low magnification indicates localizations of GFP + patches. Dotted areas in f indicate GFP patches in GFP/dnMAMl-electroporated brains displaying high levels of Cxcl12 mRNA ( n =6 for each group). ( g , h ) GFP, EdU and Iba1 labelling in electroporated embryos injected with EdU (3 h). Boxed areas indicate the region of interest in electroporated patches from GFP ( g ) and GFP/dnMAMl ( h ) embryos. ( i ) Quantifications of Iba1 + cells (mean±s.e.m., n =7 brains for each group), while percentages±s.e.m. of Iba1/EdU + cells are provided in j ( n =5 for each group). ( k ) Total number of Iba1 + cells in GFP/dnMAMl-electroporated patch performed on Gfap Cre Cxcl12 f/+ and Gfap Cre Cxcl12 f/f mice, while quantifications are shown in l (means±s.e.m., n =3 for each group). Scale bar represents 100 and 10 μm for insets in e . A two-tailed t -test was used to assess statistical significance: ** P <0.01, *** P <0.001. Full size image Neurogenesis promotes microglia recruitment during cerebral cortex development To functionally validate the close relationship between BP generation and microglia recruitment into the VZ/SVZ, we next assessed whether defective neurogenesis might influence Iba1 + cell recruitment or positioning into the cerebral cortex. We first analysed Gfap Cre /β-Catenin Ex3 mice owing to their propensity to express a stabilized and constitutive active form of β-catenin in cortical RG leading to a dramatic impairment of Tbr2 + cell generation [29] , [30] . At E14.5 the expression of Cxcl12 was almost completely abolished in the cortical SVZ of Gfap Cre /β-Catenin Ex3 mice ( Fig. 5a,b ), while it was preserved at the cortical–striatal notch and within meninges—which express Cxcl12 at high levels [9] —two regions in which the CRE-mediated recombination of β-Catenin Ex3 allele does not occur. At the same time point, the number of microglia was significantly reduced in the VZ/SVZ ( Fig. 5c–e ). To rule out the possibility that the deletion of β-catenin might affect endothelial cells—in which β-catenin is involved in controlling vascular remodelling [31] —that might contribute to influence microglia migration, we analysed CD31 + endothelial cells in Gfap Cre /β-Catenin Ex3 mice. CD31 + cells were unaffected in the cortical wall of Gfap Cre /βCatenin Ex3 mice ( Supplementary Fig. 7a,b ). 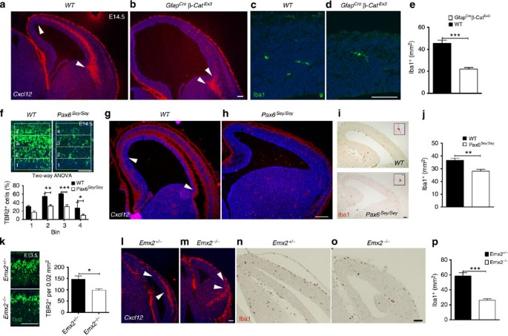Figure 5: Microglia recruitment is affected in transgenic mice displaying altered neurogenesis. (a,b)Cxcl12 in situhybridization on (E14.5)WTandGfapCreβ-CateninEx3mice (arrowheads indicate the extension ofCxcl12+domains in the developing cortical wall). (c–e) Iba1 labelling ofWTandGfapCreβ-CateninEx3mice and their quantifications into the cerebral cortex (mean±s.e.m.,n=3 brains for each group). (f) Quantifications of Tbr2+cells in laminar bins encompassing the VZ/SVZ of WT andPax6Sey/Seymice (E14.5, means±s.e.m.,n=3 for each group). (g–j)Cxcl12 in situhybridizations inWTandPax6Sey/Seymice and Iba1 labelling and quantification (mean±s.e.m.,n=3 brains for each group). (k) Quantification of Tbr2+cells in caudal cortical walls ofEmx2+/−andEmx2−/−mice (E13.5, mean±s.e.m.). (l,m)Cxcl12, byin situhybridization in caudal sections ofEmx2+/−andEmx2−/−mice. (n–p) Iba1 labelling and quantifications onEmx2+/−andEmx2−/−(mean±s.e.m.,n=3 brains for each group). Scale bar represents 100 μm. A two-tailedt-test was used to assess statistical significance: *P<0.05, **P<0.01, ***P<0.001. Figure 5: Microglia recruitment is affected in transgenic mice displaying altered neurogenesis. ( a , b ) Cxcl12 in situ hybridization on (E14.5) WT and Gfap Cre β-Catenin Ex3 mice (arrowheads indicate the extension of Cxcl12 + domains in the developing cortical wall). ( c – e ) Iba1 labelling of WT and Gfap Cre β-Catenin Ex3 mice and their quantifications into the cerebral cortex (mean±s.e.m., n =3 brains for each group). ( f ) Quantifications of Tbr2 + cells in laminar bins encompassing the VZ/SVZ of WT and Pax6 Sey/Sey mice (E14.5, means±s.e.m., n =3 for each group). ( g – j ) Cxcl12 in situ hybridizations in WT and Pax6 Sey/Sey mice and Iba1 labelling and quantification (mean±s.e.m., n =3 brains for each group). ( k ) Quantification of Tbr2 + cells in caudal cortical walls of Emx2 +/− and Emx2 −/− mice (E13.5, mean±s.e.m.). ( l , m ) Cxcl12 , by in situ hybridization in caudal sections of Emx2 +/− and Emx2 −/− mice. ( n – p ) Iba1 labelling and quantifications on Emx2 +/− and Emx2 −/− (mean±s.e.m., n =3 brains for each group). Scale bar represents 100 μm. A two-tailed t -test was used to assess statistical significance: * P <0.05, ** P <0.01, *** P <0.001. Full size image Furthermore, in Pax6 Sey mice we found, at E14.5, a significant reduction of Tbr2 + cells in the cortical VZ/SVZ ( Fig. 5f ), as expected in the absence of Cxcl12 transcripts in the SVZ ( Fig. 5g,h ) [6] and, above all, a significant reduction of microglia in the cerebral cortex ( Fig. 5i,j ). Since Emx2 is a transcription factor involved in the maintenance of RG self-renewal [32] , [33] , we then investigated microglia in Emx2 −/− mice that are characterized by a significant perturbation of neurogenesis in the caudal telencephalon [33] . Interestingly, the number of Tbr2 + cells was significantly reduced in the posterior cerebral cortex of Emx2 −/− brains ( Fig. 5k ) and such reduction was paralleled by a substantial reduction of Cxcl12 ( Fig. 5l,m ). Consistently, we detected a significant depletion of microglia in same regions of the brain ( Fig. 5n–p ); however, no alteration of CD31 + endothelial cells was found ( Supplementary Fig. 7c,d ). Cell death in the developing forebrain triggers microglia proliferation We next explored whether we could attribute the above-mentioned results to the recently described capability of microglia to regulate the number of neural precursor via phagocytosis [14] , [34] . We, thus, assessed whether a functional derangement of RG might, in turn, influence microglia into the VZ/SVZ. E14.5 embryos were electroporated with the suicide gene Thymidine Kinase ( TK ) and treated with Ganciclovir (GCV) at different time points thereafter, that is, at E14.7, E15.5 and E16.2. Activated Caspase3 + cells (Casp3a) were significantly increased in TK (+GCV) compared with GFP control mice ( Fig. 6a–c ). Increased rate of cell death was paralleled by increased number of microglia displaying a phagocytic cell morphology ( Fig. 6d,e ). The absolute number of Iba1 + cells as well as percentages of proliferating Iba1/EdU + cells were increased ( Fig. 6f–i ). Along the same lines, we explored FoxG1 −/− mice that show increased rates of neuronal cell death during neurogenesis [35] . Although FoxG1 −/− mice also displayed several morphological defects, involving the loss of basal ganglionic eminence specification [36] , and defective cortical arealization [37] , we found that in these mice the number of Iba1 + cells was substantially increased into the rudimental cerebral cortex and, above all, they displayed cell morphology reminiscent of phagocytic cells ( Fig. 6h,i ). 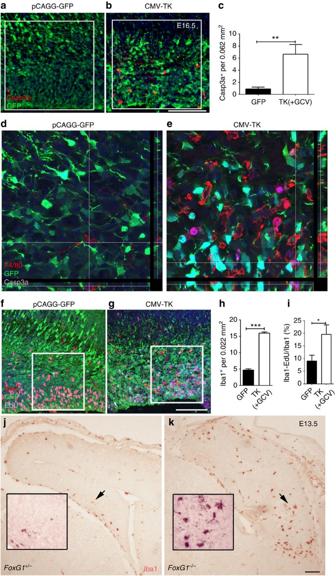Figure 6: Increased cell death rates into the VZ/SVZ-triggered microglia proliferation. (a,b) GFP and Casp3a labelling in E16.5 brains electroporated either with GFP (a) or TK plasmids and then injected with GCV (b). (c) Quantifications of Casp3a+cells in boxed areas (mean±s.e.m.,n=6 brains for each group). (d,e) Confocal stacks of F4/80, GFP and Casp3a cells in GFP (d) and TK (+GCV;e) electroporated E16.5 embryos. (f,g) Iba1, GFP and EdU (3 h pulse) labelling in GFP and TK (+GCV) mice, to score proliferating microglia. (h,i) Quantifications of total Iba1+cells (mean±s.e.m.) and percentages of Iba1/EdU+cells (±s.e.m.,n=6 brains for each group). (j,k) Iba1 labelling in E13.5 FoxG1+/−(j) and FoxG1−/−(k) brains (insets in both panels show high magnifications of Iba1+cells into cortical fields,n=3 brains for each group). Scale bar represents 100 μm. A two-tailedt-test was used to assess statistical significance: *P<0.05, **P<0.01, ***P<0.001. Figure 6: Increased cell death rates into the VZ/SVZ-triggered microglia proliferation. ( a , b ) GFP and Casp3a labelling in E16.5 brains electroporated either with GFP ( a ) or TK plasmids and then injected with GCV ( b ). ( c ) Quantifications of Casp3a + cells in boxed areas (mean±s.e.m., n =6 brains for each group). ( d , e ) Confocal stacks of F4/80, GFP and Casp3a cells in GFP ( d ) and TK (+GCV; e ) electroporated E16.5 embryos. ( f , g ) Iba1, GFP and EdU (3 h pulse) labelling in GFP and TK (+GCV) mice, to score proliferating microglia. ( h , i ) Quantifications of total Iba1 + cells (mean±s.e.m.) and percentages of Iba1/EdU + cells (±s.e.m., n =6 brains for each group). ( j , k ) Iba1 labelling in E13.5 FoxG1 +/− ( j ) and FoxG1 −/− ( k ) brains (insets in both panels show high magnifications of Iba1 + cells into cortical fields, n =3 brains for each group). Scale bar represents 100 μm. A two-tailed t -test was used to assess statistical significance: * P <0.05, ** P <0.01, *** P <0.001. Full size image We next investigated the molecular mechanism underlying the proliferation of microglia in TK (+GCV) embryos. We screen several neuronal- and glial cell- (including RG) secreted molecules that might have the potential to induce microglia proliferation. Among them, we concentrated on MIF [38] , [39] , since it has been consistently shown that this cytokine can modulate myeloid cell proliferation by binding to the CD74 receptor [40] . By in situ hybridization we detected MIF mRNA in germinal niches of the developing cerebral cortex at E12.5, E14.5, E16.5 and E18.5. Starting from E14.5, we also found scattered neurons, located within the cortical plate, expressing MIF transcripts. Interestingly, MIF was expressed in the cortical VZ along a medial high to lateral low gradient ( Fig. 7a ). Real-time PCR on CD133 + and CD45 low /CD11b + -sorted cells from E14.5 forebrains confirmed that MIF was expressed by RG and also by microglia ( Fig. 7b ). CD74 expression was confirmed in whole cortical extracts from E14.5 brains and in CD45 low /CD11b + -sorted cells, but not in CD133 + -sorted cells ( Fig. 7c ). We confirmed that MIF can modulate microglia cell proliferation by electroporating vectors encoding MIF at E14.5. ( Fig. 7d ). Iba1/XdU + cells were significantly increased in cortices receiving MIF, as compared with untreated and GFP controls ( Fig. 7e ). We next blocked MIF/CD74 interaction by injecting, into the ventricular cavity of E14.5 embryos, the allosteric MIF inhibitor p425 (1 μl, 0.5 mM), a molecule known to interfere with binding of MIF to the CD74 receptor [41] . Because p425 shows a brilliant blue tint in colour, we efficiently monitored its brain penetration. Proliferating microglia were scored at E15.5 by labelling embryos with 5-ethynyl-2′-deoxyuridine (EdU) for 12 h. MIF blockade significantly reduced percentages of Iba1/EdU + cells, if compared with embryos receiving vehicle only (sham: 25.7%±2; p425 12.5%±2, n =3 for each group, mean percentages±s.d., P <0.001, two-tailed t -test). To analyse whether or not increased rates of microglia proliferation in TK (+GCV) embryos was depending on MIF, we first analyse MIF mRNA expression in embryos injected with TK (+GCV). By in situ hybridization, we observed a substantial increment of MIF mRNA levels in embryos receiving TK (+GCV; Fig. 7h,i ) compared with embryos receiving the GFP plasmid only ( Fig. 7f,g ). We next performed MIF blockage in TK (+GCV) brains by co-injecting p425 at the time of electroporation. Interestingly, the numbers of dying cells in TK (+GCV) mice was not altered by the treatment with p425 ( Fig. 7j,k ), while microglia proliferation was significantly reduced in embryos receiving TK (+GCV) along with p425 ( Fig. 7l–n ). 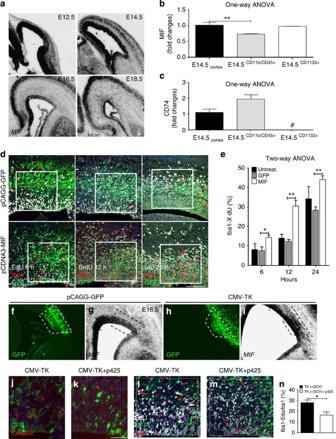Figure 7: MIF regulates proliferation of cortical microglia. (a)In situhybridization forMIFat E12.5, E14.5, E16.5 and E18.5 (n=3 brains for each group). Real-time PCR forMIFandCD74were performed on E14.5 whole cortical extracts, E14.5-sorted CD45low/CD11b+cells and E14.5-sorted CD133+cells. Normalized fold changes (means±s.e.m.) are shown inb,c(n=3 for each group). (d) Confocal stacks of sections electroporated with GFP (upper row) or MIF (lower row), and then injected with EdU, BrdU and IdU (6, 12 and 24 h) and finally labelled for GFP, Iba1 and the S-phase tracer. (e) Iba1/XdU+cells (percentages±s.e.m.) in boxed areas (n=3 brains for each group). Embryos electroporated with the GFP (f,g) or with GFP/TK (+GCV;h,i) labelled for GFP (f,h) to identify electroporated patches and forMIF, byin situhybridization (g,i;n=4 brains for each group). (j,k) GFP and Casp3a labelling on E16.5 embryos electroporated either with GFP/TK (+GCV) or GFP/TK(+GCV) and receiving p425 (0.5 mM). (l–n) Iba1(red), GFP (green) and EdU (white) labelling and quantifications on embryos electroporated either with GFP/TK (+GCV) or GFP/TK (+GCV) and p425 (0.5 mM;n=3 for each group). One-way and two-way ANOVA tests with Bonferroni post test and a two-tailedt-test were used to assess statistical significance: *P<0.05, **P<0.01, ***P<0.001. Scale bar represents 100 μm. Figure 7: MIF regulates proliferation of cortical microglia. ( a ) In situ hybridization for MIF at E12.5, E14.5, E16.5 and E18.5 ( n =3 brains for each group). Real-time PCR for MIF and CD74 were performed on E14.5 whole cortical extracts, E14.5-sorted CD45 low /CD11b + cells and E14.5-sorted CD133 + cells. Normalized fold changes (means±s.e.m.) are shown in b , c ( n =3 for each group). ( d ) Confocal stacks of sections electroporated with GFP (upper row) or MIF (lower row), and then injected with EdU, BrdU and IdU (6, 12 and 24 h) and finally labelled for GFP, Iba1 and the S-phase tracer. ( e ) Iba1/XdU + cells (percentages±s.e.m.) in boxed areas ( n =3 brains for each group). Embryos electroporated with the GFP ( f , g ) or with GFP/TK (+GCV; h , i ) labelled for GFP ( f , h ) to identify electroporated patches and for MIF , by in situ hybridization ( g , i ; n =4 brains for each group). ( j , k ) GFP and Casp3a labelling on E16.5 embryos electroporated either with GFP/TK (+GCV) or GFP/TK(+GCV) and receiving p425 (0.5 mM). ( l – n ) Iba1(red), GFP (green) and EdU (white) labelling and quantifications on embryos electroporated either with GFP/TK (+GCV) or GFP/TK (+GCV) and p425 (0.5 mM; n =3 for each group). One-way and two-way ANOVA tests with Bonferroni post test and a two-tailed t -test were used to assess statistical significance: * P <0.05, ** P <0.01, *** P <0.001. Scale bar represents 100 μm. Full size image In conclusion, our data support the notion that MIF is acting as a mitogenic cue for microglia residing within the developing cerebral cortex that upregulates when tissue damage occurs. BP number is reduced in mice lacking Csf-1R We explored whether or not microglia might contribute to the proper generation of cortical BP by analysing embryos lacking Csf-1R , a receptor known to be essential for microglia development ( Fig. 8d,e ) [11] , [42] . At E13.5, the number of Tbr2 + cells was slightly, but significantly, reduced in the inner SVZ from CMV Cre Csf-1R flox/flox mice ( Fig. 8a–c ). At E17.5, Tbr2 + cells were further depleted in the SVZ of CMV Cre Csf-1R flox/flox mice ( Fig. 8d–h ) and such reduction was mirrored by a reduction of pH3 + mitoses in the SVZ ( Fig. 8i–k ). The number of Casp3a + cells, however, did not increase in the cerebral cortex of CMV Cre Csf-1R flox/flox mice at E13.5 (WT: 1.6±0.4 cells per section; knockout (KO): 2.0±0.8 cells per section; mean±s.d., P =0.17, two-tailed t -test) as well as at E17.5 (WT:1.9±0.4 cells per section; KO: 2.6±0.8 cells per section; mean±s.d., P =0.08, two-tailed t -test. ), thus suggesting that the presence of microglia into germinal niches of the brain is contributing to the homeostasis/maintenance of an appropriate BP pool. 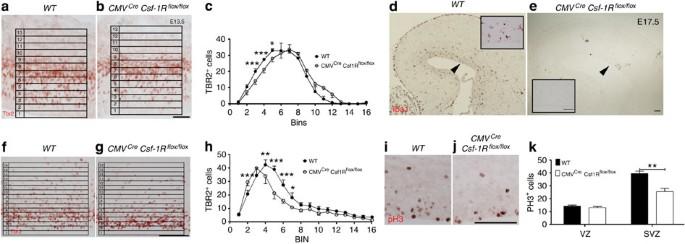Figure 8: Tbr2+cells are diminished in the cerebral cortex ofCsf-1Rconditional knockout mice. (a–c) Tbr2 labelling and quantifications (means±s.e.m.) performed on cortical sectors 300 μm wide, subdivided into bins of 20 μm in height, inWT(a) andCMVCreCsf-1Rflox/flox(b) mice at E13.5 (n=3 for each group). (d,e) Iba1 labelling on E17.5 coronal sections fromWTandCMVCreCsf-1Rflox/floxmice. Insets in both panels show high-magnification views of the VZ/SVZ. (f–h) Tbr2 labelling and quantifications (means±s.e.m.) performed in cortical sectors 400 μm wide, subdivided into bins of 20 μm in height of E17.5WTandCMVCreCsf-1Rflox/floxmice. (i–k) PH3 labelling and quantifications (means±s.e.m.) in the VZ/SVZ of E17.5WT(i) andCMVCreCsf-1Rflox/flox(j) mice (n=3 brains for each genotype). Scale bar represents 100 μm. A two-tailedt-test was used to assess statistical significance: *P<0.05, **P<0.01, ***P<0.001. Figure 8: Tbr2 + cells are diminished in the cerebral cortex of Csf-1R conditional knockout mice. ( a – c ) Tbr2 labelling and quantifications (means±s.e.m.) performed on cortical sectors 300 μm wide, subdivided into bins of 20 μm in height, in WT ( a ) and CMV Cre Csf-1R flox/flox ( b ) mice at E13.5 ( n =3 for each group). ( d , e ) Iba1 labelling on E17.5 coronal sections from WT and CMV Cre Csf-1R flox/flox mice. Insets in both panels show high-magnification views of the VZ/SVZ. ( f – h ) Tbr2 labelling and quantifications (means±s.e.m.) performed in cortical sectors 400 μm wide, subdivided into bins of 20 μm in height of E17.5 WT and CMV Cre Csf-1R flox/flox mice. ( i – k ) PH3 labelling and quantifications (means±s.e.m.) in the VZ/SVZ of E17.5 WT ( i ) and CMV Cre Csf-1R flox/flox ( j ) mice ( n =3 brains for each genotype). Scale bar represents 100 μm. A two-tailed t -test was used to assess statistical significance: * P <0.05, ** P <0.01, *** P <0.001. Full size image Despite recent progress in elucidating the function of microglia in the healthy and pathological central nervous system, still the molecular mechanism controlling microglia recruitment into the developing brain is largely unknown. Here we show, using several in vivo functional approaches, that microglia recruitment into the cortical VZ/SVZ is dependent on Cxcl12 -expressing BP cells. Indeed, we demonstrated that primary microglia cell cultures [43] and cortical microglia express both Cxcl12 receptors, a feature necessary for BP expressing Cxcl12 (refs 6 , 44 , 45 ) to attract microglia into the VZ/SVZ. Accordingly, the downregulation of Cxcl12 in FoxG1 Cre /Tbr2 flox/flox mice reduced ~40% the number of CxcR4/CxcR7/CaB + neurons migrating into the cortex [5] , and a 25% reduction of microglia into the cortex was observed in Gfap Cre /Tbr2 flox/flox mice. In line with these results, the ectopic expression of either Tbr2 or Cxcl12 substantially increased the number of microglia within the electroporated areas. Furthermore, the injection of AMD3100—a blocker of Cxcl12/CxcR4 interaction [21] —as well as the constitutive inactivation of CxcR4 and the conditional inactivation of Cxcl12 ( Gfap Cre Cxcl12 flox/flox ) caused a significant reduction of cortical microglia cells. To further sustain the finding that BPs are involved in the recruitment of microglia at the VZ/SVZ, we examined transgenic mice in which the proper generation of BP within the developing cerebral cortex is impaired. In mice carrying a constitutive active form of β-Catenin [46] in RG—a genetic alteration that prevents RG to acquire the BP phenotype and to differentiate into Tbr2 + cells [29] , [30] , [47] —the reduction of BP affected Cxcl12 expression in the SVZ and the number of microglia was reduced to ~60%. In Pax6 Sey/Sey mice, carrying a null allele for the transcription factor Pax6 , Tbr2 + cells were greatly reduced, Cxcl12 expression was suppressed into the SVZ [6] and a significant reduction of microglia was observed. In mice lacking Emx2 —a transcription factor promoting RG proliferation in the occipital cortex [48] —the number of Tbr2 + cells was reduced to 30% and the expression of Cxcl12 was greatly impaired. In the same mice, the reduction of Cxcl12 was paralleled by a 30% reduction of microglia in the occipital cortex. On the other hand, the inhibition of Notch signalling in RG increased both BP cells and the expression of Cxcl12 in the developing cortex, a finding accompanied by a threefold increase in the microglia number. Nonetheless, we observed that microglia cells were not completely eliminated in all the above-mentioned mutant mice. This might suggest the existence of additional, still unknown, factors that might contribute to microglia positioning/recruitment in the developing forebrain. Some hypotheses can be put forward. Embryonic leptomeninx—that express Cxcl12 (ref. 9 ) to promote the development of Cajal–Retzius cells [49] —are not affected in our mutant mice, thus suggesting that they might per se contribute to attract circulating microglia. Owing to the fact that ~20% of the mid-end gestational cortical microglia is actively proliferating [15] , we cannot exclude that cell proliferation represents a rescue mechanism aimed at balancing microglia depletion occurring as a consequence of Cxcl12 reduction. Apart from the existence of additional sources of Cxcl12 in the developing brain, we cannot rule out the possibility of the existence in the developing brain of microglia progenitors, able to proliferate in order to replenish the microglia cell pool as occurs in pathological conditions determining microglia depletion in the adult brain [50] . Interestingly, we observed a Cxcl12-independent increased rate of microglia proliferation in embryos receiving the TK suicide gene along with GCV treatment; as such, we found an increased number of microglia in areas harbouring cells undergoing apoptosis. Thus, we might speculate that the ability of microglia to regulate neural precursor homeostasis by removing dying cells during forebrain development might be also retained in the adult brain as a rescue mechanism under pathological conditions. How about mitotic cues promoting microglia proliferation? We found that MIF , expressed by CD133 + RG, can stimulate microglia proliferation by acting on CD74. Remarkably, increased levels of MIF have been found in microglia-driven inflammatory reactions occurring in neurodegenerative diseases (that is, multiple sclerosis, stroke and Parkinson’ disease) [51] and in microglia cells associated to gliomas [52] . All together, these data further support the emerging concept that chemokines and cytokines may play not only detrimental but also protective roles. This appears to be much more depending on target cells as well as environmental features [53] . A growing number of studies have suggested that activated microglia modulates adult neurogenesis [54] , [55] , [56] , even under pathological conditions such as in multiple sclerosis [57] and stroke [58] . On one hand, in the embryonic SVZ, microglia seems to be able to limit the number of BP [14] : pharmacological manipulations increasing the number of microglia showing an M1 phenotype causes a substantial reduction of Tbr2 + cells, while a decrease in microglia or skewing microglia towards the M2 phenotype leads to an increase in the number of Tbr2 + cells [14] . On the other hand, recent evidence suggests that cytokines released by activated microglia might enhance both neurogenesis and oligodendrogenesis in the early postnatal SVZ [34] . To better understand the reason of these controversial results, we thus measured BP in Csf-1R null mice that are microglia-free. The constitutive inactivation of Csf-1R causes significant alterations of brain morphology at postnatal stages, such as: a reduction in cortical thickness, the underdevelopment of olfactory bulbs [42] , a distortion of the hippocampus and a reactive astrogliosis. However, such alterations are not affecting the forebrain during embryonic development. A finding attributable to the fact that Csf-1R is expressed in the adult brain not only by myeloid cells but also by few cortical and hippocampal neurons [59] , while it is expressed only by microglia during brain development [60] . Consistently with this hypothesis, we found that Tbr2 + BPs were slightly, but significantly, reduced in Csf-1R null mice at E13.5 and at E17.5. This observation suggests that in the developing brain microglia can certainly contribute to removing progenitor cells—as previously shown by in ref. 14 and confirmed by our results in TK-electroporated mice—but its primary role is to support neurogenesis. Nevertheless, we cannot exclude the possibility that depending on the state of activation, different microglia subpopulations might exert still unrevealed different functional roles on proliferating progenitors. In conclusion, we demonstrated that microglia clustering into germinal niches of the developing cortex is largely dependent on BP expressing Cxcl12 and that the mutual bidirectional relationship between these two cell types is vital to protect the developing cerebral cortex from unexpected damage impairing the proper proliferation and cortical positioning of neural precursors. Animals Mice were maintained under pathogen-free conditions at San Raffaele Hospital mouse facility (Milan, Italy). All efforts were made to minimize animal suffering and to reduce the number of mice used in accordance with the European Communities Council Directive of 24 November 1986 (86/609/EEC). All animal experimental protocols were approved by the Ethics Review Committee for Animal Experimentation of the Italian Ministry of Health. Procedures were performed according to the guidelines of the Institutional Animal Care and Use Committee of the San Raffaele Scientific Institute (protocol number 727/2011). Cx3Cr1-GFP mice [16] were provided by Dr Verderio (University of Milan, Italy); Tbr2 flox/flox conditional mice [61] were provided by Dr Broccoli (San Raffaele Scientific Institute, Italy); Gfap Cre mice [62] were obtained from Jackson Laboratories; β-Catenin Ex3 mice [46] were provided by Dr Taketo (Kyoto University, Japan); Emx2 −/− and Pax6 Sey mice [63] , [64] were provided by Dr Nicolis (University of Bicocca, Italy); FoxG1 −/− mice [65] were provided by Dr McConnel (Stanford University, USA); CMV Cre and Csf-1R flox/flox (ref. 66 ) were purchased from the Jackson Laboratory; CxcR4 −/− (ref. 67 ) mice were provided by Dr Bianchi (San Raffaele Scientific Institute); and Cxcl12 flox/flox conditional mice [68] were purchased from the Jackson Laboratory. Transgenic mice were backcrossed on C57Bl/6 (Charles River) mice and were genotyped as previously described [4] , [29] , [48] , [65] . In utero electroporation was carried out on C57Bl/6 mice. At noon the vaginal plug date was day 0.5 in timed pregnancies. S-phase labelling was carried out as previously described [69] . Depending on the protocol of administration, pregnant dams received single or multiple injections of S-phase tracers—that is, 5-bromodeoxyuridine (BrdU), 5-Iododeoxyuridine (IdU) (Sigma, St. Louis, MO, USA) and EdU (Invitrogen, Carlsbad, CA, USA) at the concentration of 100 mg kg −1 . Pregnant females were killed by cervical dislocation at appropriate time points and brains were collected in ice-cold PBS as previously described [69] . Brains were fixed in 4% Paraformaldehyde (Sigma) in PBS, pH 7.2 for 12 h at +4 °C, cryoprotected in PBS-30% Sucrose (Sigma) and then embeded in OCT inclusion media. Samples were stored at −80 °C before processing. Human fetal tissues were collected from patients who requested pregnancy termination and autopsy diagnostic procedures. All procedures were approved by the local research ethical committees and Research services division of the University of Cambridge and Addenbrooke’s Hospital in Cambridge and by Ethics Committee of San Paolo Hospital (Milan). Immunofluorescence and in situ hybridization Briefly, the sections (12 μm) were washed three times, 5 min each in PBS, and the blockage of nonspecific binding was performed by using the following mix: PBS 1 × /FBS 10%/BSA 1 mg ml −1 Triton × 100 0.1%, for 1 h at room temperature. In the case of BrdU, IdU detections, DNA was depurinated to make epitopes accessible to antibodies by incubating slides in HCl 2N for 30′. Slides were then rinsed in borate buffer (0.1 M, pH 8.5) for 10 min at room temperature. Antibodies were diluted in blocking mix and incubated at +4 °C overnight as suggested by the manufacturer’s instructions. The following day, sections were rinsed in PBS for 5 min, three times, and fluorescent secondary antibodies (Alexafluor conjugated) diluted in blocking mix, were applied according to the manufacturer’s instructions. Slides were washed three times in PBS for 5 min and incubated in Hoechst 33342 for nuclei counterstaining. When necessary, antigens retrieval was performed by boiling samples in 10 mM sodium citrate (pH 6) for 5 min. The following antibodies were used: rabbit α-CxcR4 (Novus) 1:100; rabbit α-Iba1 (Wako) 1:400; rabbit α-Tbr2 (Abcam) 1:500; chicken α-GFP (Abcam) 1:500; rabbit α-pH3 (Cell Signaling) 1:200; rat α-CD206 (BD) 1:50; rabbit α-Ki67 (Novocastra) 1:100; rabbit α-CaB (Swant) 1:500; rat α-CD31 (BD) 1:100; rat α-BrdU (Abcam) 1:500; mouse α-IdU (BD) 1:75; rat α-CD45 (BD) 1:100; rabbit α-Casp3a (BD) 1:400; mouse α-F4/80 (Abcam) 1:200; rabbit α-Blbp (Millipore) 1:700; and click-it EdU alexafluor 647 imaging reagent (Invitrogen). Appropriate fluorophore-conjugated secondary antibodies (Alexa-Fluor 488, 546 and 633 Molecular Probes) were applied according to the manufacturers’ instruction. Immunohistochemistry was carried out as previously described [57] . Briefly, slices were incubated in H 2 O 2 3% for 20 min before adding the blocking mix. Antibodies were diluted in blocking mix and incubated at +4 °C overnight, as described above. The following day, sections were washed in PBS three times, and the biotin-conjugated secondary antibody (Vector labs, Milan, Italy) was applied for 2 h. Then sections were washed before adding the avidin-HRP reagent (Vector). Signals were revealed by incubating slices with 3-amino-9-ethylcarbazole (AEC, Sigma) solution. In situ hybridization was performed as previously described [48] . Briefly, 12-μm-thick brain cryosections were post-fixed 15 min in 4% paraformaldehyde and then washed three times in PBS. Slides were incubated in 0.5 mg ml −1 of Proteinase K in 100 mM Tris–HCl (pH 8) and 50 mM EDTA for 10 min at 30 °C. This was followed by 15 min in 4% paraformaldehyde. Slices were then washed three times in PBS before receiving H 2 O washes. Sections were incubated in Triethanolamine 0.1 M (pH 8) for 5 min, and then 400 μl of acetic anhydride was added three times for 5 min each. Finally, the sections were rinsed in H 2 O for 2 min and air-dried. Hybridization was performed overnight at 60 °C with P [32] riboprobes at a concentration ranging from 10 6 to 10 7 counts per minute (c.p.m.) per slide. The following day, the sections were rinsed in SSC 5 × for 5 min and then washed in Formamide 50% SSC 2 × for 30 min at 60 °C. Then the slides were incubated in Ribonuclease-A (Roche) 20 mg ml −1 in 0.5 M NaCl, 10 mM Tris-HCl (pH 8) and 5 mM EDTA 30 min at 37 °C. The sections were further washed in Formamide 50% SSC 23 for 30 min at 60 °C and then the slides were rinsed two times in SSC 2 × . Finally, the slides were dried by using Ethanol series. NTB emulsion (Carestream) was applied in a dark room, according to the manufacturer’s instructions. After 1 week, the sections were developed in the dark room, counterstained with Hoechst 33342 and mounted with DPX (BDH) mounting solution. Digoxigenin in situ hybridization on frozen sections were performed as previously reported [33] . The following probes were used: Cxcl12 (kind gift of Dr Broccoli, San Raffaele Institute, Milan, Italy), Ttr was PCR-amplified on the basis of Genebank DT00071, nt 13-1484, MIF was PCR-amplified on the basis of Gene bank NM_010798, MIF PCR-amplified on the basis of Genebank NM_010798, nt 20–300. Light (Olympus, BX51 with × 4 and × 20 objectives) and confocal (Leica, SP5 with × 40 objective) microscopy was performed to analyse tissue and cell staining. Analysis was performed by using the Leica LCS lite software and the Adobe Photoshop CS software. Quantification of Iba1 + cells in E14.5 and E18.5 WT brains was carried out by the Stereo Investigator v 3.0 software (MicroBrightField Inc., Colchester, VT, USA). Flow cytometry and cell sorting Cell suspensions were made from E14.5 and E15.5 forebrains. Briefly, tissues were cut into small pieces and incubated in ice-cold HBSS 1 × , Glucose 0.6%, Hepes pH 7.4, 5 mM. Upon mechanical dissociation, cell suspensions were filtered through 40-μm cell strainer and then washed three times in HBSS 1 × and stained with the following monoclonal antibodies: α-CD11b PE-Cy7 (BD), α-CD45 FITCH (BD), α-CxcR4 APC (BD), α-CD133 APC (eBioscience) and α-Ly6C APC (BD). Flow cytometry studies were performed using a Canto-DIVA (Becton Dickinson) and subsequently analysed using the FCS-Express software ( De Novo ). Cell sorting was performed by using MoFlow sorter. Approximately 10–20 × 10 5 MG cells were obtained from 15 brains and 2 × 10 6 CD133 + cells were obtained from 10 brains. Primary microglia cultures and chemotactic assay Mouse primary microglia were raised P2 C57BL6/j pups, as follows. Brains were excised and placed in ice-cold HBSS. Cortices were removed, meninges were pulled off and the remaining tissue was minced with forceps. Neural Dissociation Kit (P) (Miltenyi-Biotec) was used to obtain a single-cell suspension from minced tissue. Mixed glial cells were then plated at 1 × 105 cells per ml in T75 Flask and cultured in DMEM supplemented by 10% fetal bovine serum (Invitrogen), 1% GlutaMAX (Invitrogen) and 1% penicillin/streptomycin in a 5% CO 2 /37 °C incubator. The medium was changed every 3 days, for a total of 14 days. Microglia cells were then collected by vigorous shaking of flasks, for at least 5–10 min and percentages of Iba1+ cells were evaluated with flow cytometry. Chemotaxis assay: Cxcl12-mediated microglia recruitment was tested in vitro using Cxcl12 (Invitrogen) with or without the Cxcl12/CxcR4 antagonistAMD3100 (Sigma-Aldrich). Transwell inserts (pore size, 8 μm, BD Biosciences) and 24-well culture plates (Corning Costar) were used to that mean. Cell-free conditioned medium alone or with increasing Cxcl12 concentration (10, 100 and 200 ng ml −1 , Cxcl12 200 ng ml −1 AMD3100 1 ng ml −1 ) were placed in lower chambers. Microglia were placed in upper chambers at 6 × 105 cells per ml in the serum-free medium. The transwell plates were incubated for 12 h at 37 °C. Migrated microglia cells were led to adhere to pre-coated p-lysine in 12-mm coverslips. Standard immunostaining for Iba was then performed. In utero electroporation and drug injections The following plasmids were injected into the ventricular cavity of E14.5 forebrains (Charles River Italy): pCAGG-GFP (0.1 μg μl −1 ), pCAGG-Cxcl12 4 (1 μg μl −1 ), pCAGG-Tbr2 4 (0.6 μg μl −1 ), pCAGGS-dnMAMl.eGFP [26] (2.5 μg μl −1 ), pCDNA3-MIF (1 μg μl −1 ) and pCDNA3-TK (1 μg μl −1 ). Plasmids were mixed with 0.01% Fast green (Sigma), and 1–2 μl of each DNA mix were injected into the ventricle through a fine-glass capillary. Electrodes (Tweezertrodes, BTX Harvard Apparatus, Holliston, MA, USA) were placed flanking the ventricular region of each embryo, covered by a drop of PBS and pulsed four times at 50 V for 50 ms, separated by intervals of 950 ms, with a square wave electroporator (ECM 830, BTX Harvard Apparatus). Then, the uterine horn was placed back into the abdominal cavity filled with warm PBS 1 × . Embryos were left to develop in utero for 48 h and then administered with S-phase tracers (EdU, IdU and BrdU accordingly each experimental paradigm) as above described. In some experiments we included embryos only receiving surgery, that are referenced as untreated. For blocking of Cxc12/CxcR4 interaction, 1 μl of AMD3100 solution (12.6 mM; Sigma) or PBS was injected into the lateral ventricle at E12.5 and the embryos were left to develop in utero for 20 h. For blocking MIF/CD74 interaction, 1 μl of p425 (ref. 41 ; 0.5 mM) or PBS was injected in the lateral ventricle of E14.5 and the embryos were left to develop in utero until E16.5. Real-time and standard RT–PCR Total RNA from brain tissues was extracted by using the RNeasy Mini Kit (Qiagen) according to the manufacturer’s recommendations including DNase (Promega) digestion. cDNA synthesis was performed by using the ThermoScript RT–PCR System (Invitrogen) and Random Hexamer (Invitrogen), according to the manufacturer’s instructions in final volume of 20 μl. The LightCycler 480 System (Roche) and the LightCycler 480 SYBR Green I Master Mix (Roche) were used for real-time PCR. cDNA analysis was also carried out by standard RT–PCR, performed on Bio-Rad C-1000 thermal cycler. Samples were normalized by using the housekeeping gene Histone H3 with the following primers: H3 F: 5′- GGTGAAGAAACCTCATCGTTACAGGCCTGGTAC -3′ H3 R: 5′- CTGCAAAGCACCAATAGCTGCACTCTGGAAGC -3′. Specific primers were used for gene expression analysis: CxcR4: F: 5′- GTCATCACACTCCCCTCCTGGGC -3′; R:5′- CCCTGACTGATGTCCCCCTGGC -3′ CxcR7: F: 5′- GCTTCATCAACCGCAACTACAGG -3′; R: 5′- ACCACAGGACCCAGCCGCCC -3′ MIF: F: 5′- TGGTGCCCAGAACCGCAACTAC -3′; R: 5′- GCCAGGACTCAAGCGAAGGTGG -3′ CD74: F: 5′- GCGACCTCATCTCTAACCATGAAC -3′; R: 5′- GCGAAGGCTCTCCAGTTGCAGG -3′ Iba1: F: 5′- GCAGGAAGAGAGGCTGGAGGGGATC -3′; R: 5′- CTCTTCAGCTCTAGGTGGGTCTTCGG -3′ Pax6:F: 5′- GATGGGCGCAGACGGCATGTATG -3′; R: 5′- TCTCCCCCTCCTTCCTGTTGCTG -3′ IL1β: F: 5′- CCTGTCCTGTGTAATGAAAGACGG -3′; R: 5′- TGTCCTGACCACTGTTGTTTCCC -3′ TNFα: F: 5′- GCCTCTTCTCATTCCTGCTTGTGGCAG -3′; R: 5′- GACGTGGGCTACAGGCTTGTCACTCG -3′ IFNγ: F: 5′- ACTGCCACGGCACAGTCATTGAAAGC -3′; R: 5′- CAGGTGTGATTCAATGACGCTTATGTTG -3′. Statistics Data are expressed as the mean±s.e.m. or mean±s.d. of independent experiments. Normality was assessed in each experiment by applying either Kolmogorov–Smirnov test (with Dallas–Wilkinson–Lille for P value) or Skewness test. Comparisons were made using the unpaired t -test, one-way analysis of variance (ANOVA), or two-way ANOVA followed by Bonferroni post test. Statistical tests were carried out using PRISM5.01 (GraphPad Software, La Jolla, CA, USA). A P value less than 0.05 was considered statistically significant. How to cite this article: Arnò, B. et al . Neural progenitor cells orchestrate microglia migration and positioning into the developing cortex. Nat. Commun. 5:5611 doi: 10.1038/ncomms6611 (2014).